Tight finite-key analysis for quantum cryptography Despite enormous theoretical and experimental progress in quantum cryptography, the security of most current implementations of quantum key distribution is still not rigorously established. One significant problem is that the security of the final key strongly depends on the number, M , of signals exchanged between the legitimate parties. Yet, existing security proofs are often only valid asymptotically, for unrealistically large values of M . Another challenge is that most security proofs are very sensitive to small differences between the physical devices used by the protocol and the theoretical model used to describe them. Here we show that these gaps between theory and experiment can be simultaneously overcome by using a recently developed proof technique based on the uncertainty relation for smooth entropies. Quantum Key Distribution (QKD), invented by Bennett and Brassard [1] and by Ekert [2] , can be considered the first application of quantum information science, and commercial products have already become available. Accordingly, QKD has been an object of intensive study over the past few years. On the theory side, the security of several variants of QKD protocols against general attacks has been proved [3] , [4] , [5] , [6] , [7] , [8] . At the same time, experimental techniques have reached a state of development that enables key distribution at MHz rates over distances of 100 km (refs 9 , 10 , 11 ). Despite these developments, there is still a large gap between theory and practice, in the sense that the security claims are based on assumptions that are not (or cannot be) met by experimental implementations. For example, the proofs often rely on theoretical models of the devices (such as photon sources and detectors) that do not take into account experimentally unavoidable imperfections (ref. 12 for a discussion). In this work, we consider 'prepare-and-measure' quantum key distribution protocols, like the original Bennett–Brassard 1984 (BB84) protocol [1] . Here one party prepares quantum systems (for example, the polarization degrees of freedom of photons) and sends them through an insecure quantum channel to another party who then measures the systems. To analyse the security of such protocols, the physical devices used by both parties to prepare and measure quantum systems are replaced by theoretical device models. The goal, from a theory perspective, is to make these theoretical models as general as possible so that they can accommodate imperfect physical devices independently of their actual implementation. (This approach, in the context of 'entanglement-based' protocols, also led to the development of device-independent quantum cryptography; refs 13 , 14 for recent results.) Another weakness of many security proofs is the asymptotic resource assumption, that is, the assumption that an arbitrarily large number M of signals can be exchanged between the legitimate parties and used for the computation of the final key. This assumption is quite common in the literature, and security proofs are usually only valid asymptotically as M tends to infinity. However, the asymptotic resource assumption cannot be met by practical realizations; in fact, the key is often computed from a relatively small number of signals ( M <<10 6 ). This problem has recently received increased attention and explicit bounds on the number of signals required to guarantee security have been derived [15] , [16] , [17] , [18] , [19] , [20] , [21] . In this work, we apply a novel proof technique [22] that allows us to overcome the above difficulties. In particular, we derive almost tight bounds on the minimum value M required to achieve a given level of security. The technique is based on an entropic formulation of the uncertainty relation [23] or, more precisely, its generalization to smooth entropies [22] . Compared with preexisting methods, our technique is rather direct. It therefore avoids various estimates, including the de Finetti theorem [24] and the Post-selection technique [25] , that have previously led to too pessimistic bounds. Roughly speaking, our result is a lower bound on the achievable key rate which deviates from the asymptotic result (where M is infinitely large) only by terms that are caused by, probably unavoidable, statistical fluctuations in the parameter estimation step. Moreover, we believe that the theoretical device model used for our security analysis is as general as possible for protocols of the prepare-and-measure type. Security definitions We follow the discussion of composable security in ref. 26 and first take an abstract view on QKD protocols. A QKD protocol describes the interaction between two players, Alice and Bob. Both players can generate fresh randomness and have access to an insecure quantum channel as well as an authenticated (but otherwise insecure) classical channel. (Using an authentication protocol, any insecure channel can be turned into an authentic channel. The authentication protocol will, however, use some key material, as discussed in ref. 27 .) The QKD protocol outputs a key, S , on Alice's side and an estimate of that key, Ŝ , on Bob's side. This key is usually an -bit string, where depends on the noise level of the channel, as well as the security and correctness requirements on the protocol. The protocol may also abort, in which case we set In the following, we define what it means for a QKD protocol to be 'secure'. Roughly speaking, the protocol has to, approximately, satisfy two criteria called 'correctness' and 'secrecy'. These criteria are conditions on the probability distribution of the protocol output S and Ŝ as well as the information leaked to an adversary E in general. These depend on the attack strategy of the adversary, who is assumed to have full control over the quantum channel connecting Alice and Bob, and has access to all messages sent over the authenticated classical channel. A QKD protocol is called 'correct', if, for any strategy of the adversary, Ŝ = S . It is called ɛ cor -correct, if it is ɛ cor -indistinguishable from a correct protocol. In particular, a protocol is ɛ cor -correct, if To define the secrecy of a key, we consider the quantum state ρ SE that describes the correlation between Alice's classical key S and the eavesdropper, E (for any given attack strategy). A key is called Δ-secret from E if it is Δ-close to a uniformly distributed key that is uncorrelated with the eavesdropper, that is, if where ω S denotes the fully mixed state on S . For a motivation and discussion of this particular secrecy criterion (in particular the choice of the norm) we refer to ref. 28 . A QKD protocol is called secret, if, for any attack strategy, Δ=0 whenever the protocol outputs a key. It is called ɛ sec -secret, if it is ɛ sec -indistinguishable from a secret protocol. In particular, a protocol is ɛ sec -secret, if it outputs Δ-secure keys with (1− p abort )Δ≤ ɛ sec , where p abort is the probability that the protocol aborts. (To see that this suffices to ensure ɛ sec -indistinguishability, note that the secrecy condition is trivially fulfilled if the protocol aborts.) In some applications, it is reasonable to consider correctness and secrecy of protocols separately, because there may be different requirements on the correctness of the key (that is, that Bob's key agrees with Alice's, implying that messages encrypted by Alice are correctly decrypted by Bob) and secrecy. In fact, in many realistic applications, an incorrect decoding of the transmitted data would be detected so that the data can be resent. For such applications, ɛ cor may be chosen larger than ɛ sec . However, secrecy of the protocol alone as defined above does not ensure that Bob's key is secret from the eavesdropper as well. One is thus often only interested in the overall security of the protocol (which automatically implies secrecy of Bob's key). A QKD protocol is called secure if it is correct and secret. It is called ɛ -secure if it is ɛ -indistinguishable from a secure protocol. In particular, a protocol is ɛ -secure, if it is ɛ cor -correct and ɛ sec -secret with ɛ cor + ɛ sec ≤ ɛ . Finally, the robustness, ɛ rob , is the probability that the protocol aborts even though the eavesdropper is inactive. (More precisely, one assumes a certain channel model that corresponds to the characteristics of the channel in the absence of an adversary. For protocols based on qubits, the standard channel model used in the literature is the depolarizing channel. We also chose this channel model for our analysis in the Discussion section, thus enabling a comparison to the existing results.) A trivial protocol that always aborts is secure according to the above definitions, and a robustness requirement is therefore necessary. In this work, we include the robustness ɛ rob in our estimate for the expected key rate (when the eavesdropper is inactive) and then optimize over the protocol parameters to maximize this rate. Device model Recall that Alice and Bob are connected by an insecure quantum channel. On one side of this channel, Alice controls a device allowing her to prepare quantum states in two bases, and . In an optimal scenario, the prepared states are qubits and the two bases are diagonal, for example, ={|0〉,|1〉} and ={|+〉,|−〉} with More generally, we characterize the quality of a source by its 'preparation quality', q . The preparation quality, as we will see in the following,is the only device parameter relevant for our security analysis. It achieves its maximum of q =1, if the prepared states are qubits and the bases are diagonal, as in the example above. In the following, we discuss two possible deviations from a perfect source and how they can be characterized in terms of q . First, if the prepared states are guaranteed to be qubits, we characterize the quality of Alice's device by the maximum fidelity it allows between states prepared in the basis and states prepared in the basis. Namely, we have q =−log max| 〈ψ x | ψ z 〉| 2 , where the maximization is over all states ψ x and ψ z prepared in the and basis, respectively. (In this work, log denotes the binary logarithm.) The maximum q =1 is achieved, if the basis states are prepared in diagonal bases, as is the case in the BB84 protocol. In typical optical schemes, qubits are realized by polarization states of single photons. An ideal implementation therefore requires a single-photon source in Alice's laboratory. To take into account the sources that emit weak coherent light pulses instead, the analysis presented in this paper can be extended using photon tagging [29] and decoy states [30] . This approach, although beyond the scope of the present article, can be incorporated into our finite-key analysis. (See also refs 31 , 32 , 33 for recent results on the finite-key analysis of such protocols.) Second, consider a source that prepares states in the following way: the source produces two entangled particles and then sends out one of them while the other is measured in one of two bases. The choice of basis for the measurement decides whether the states are prepared in the or basis. Together with the measurement outcome, which is required to be uniformly random for use in our protocol, this determines which of the four states is prepared. For such a source, the preparation quality is given by , where { M x } and { N z } are the elements of the positive operator-valued measurements that are used to prepare the state in the and the basis, respectively. If the produced state is that of two fully entangled qubits and the measurements are projective measurements in diagonal bases, we recover BB84 and q =1 (ref. 34 ). Sources of this type have recently received increased attention as they can be used as heralded single photon sources [35] , [36] and have applications in (device-independent) quantum cryptography [37] , [38] , [39] . On the other side of the channel, Bob controls a device allowing him to measure quantum systems in two bases corresponding to and . We will derive security bounds that are valid independently of the actual implementation of this device as long as the following condition is satisfied: we require that the probability that a signal is detected in Bob's device is independent of the basis choices ( or ) by Alice and Bob. This assumption is necessary. In fact, if it is not satisfied (which is the case for some implementations), a loophole arises that can be used to eavesdrop on the key without being detected [40] . (Remarkably, this assumption can be enforced device-independently: Bob simply substitutes a random bit whenever his device fails to detect Alice's signal. If this is done, however, the expected error rate may increase significantly.) Finally, we assume that it is theoretically possible to devise an apparatus for Bob which delays all the measurements in the -basis until after parameter estimation, but produces the exact same measurement statistics as the actual device he uses. This assumption is satisfied if Bob's actual measurement device is memoryless. (To see this, we could (in theory) equip such a device with perfect quantum memory that stores the received state until after the parameter estimation.) The assumption is already satisfied, if the measurement statistics are unaffected when the memory of the actual device is reset after each measurement. It is an open question whether this assumption can be further relaxed. Protocol definition We now define a family of protocols, Φ [ n , k , , Q tol , ɛ cor , leak EC ], which is parametrized by the block size, n , the number of bits used for parameter estimation, k , the secret key length, , the channel error tolerance, Q tol , the required correctness, ɛ cor , and the error correction leakage, leak EC . The protocol is asymmetric, so that the number of bits measured in the two bases ( n bits in the basis and k bits in the basis) are not necessarily equal [41] . These protocols are described in Box 1 . Box 1 | Protocol definition. State Preparation : The first four steps of the protocol are repeated for i =1, 2, ..., M until the condition in the Sifting step is met. Alice chooses a basis a i ∈ { , }, where is chosen with probability and with probability p z =1− p x . (These probabilities are chosen to minimize the number M of exchanged particles before Alice and Bob agree on the basis for n particles and on the basis for k particles.) Next, Alice chooses a uniformly random bit y i ∈ {0, 1} and prepares the qubit in a state of basis a i , given by y i . Alternatively, if the source is entanglement-based, Alice will ask it to prepare a state in the basis a i and record the output in y i . Distribution : Alice sends the qubit over the quantum channel to Bob. (Recall that Eve is allowed to arbitrarily interact with the system, and we do not make any assumptions about what Bob receives.) Measurement : Bob also chooses a basis, b i ∈ { , }, with probabilities p x and p z , respectively. He measures the system received from Alice in the chosen basis and stores the outcome in y ′ i ∉ {0, 1, Ø}, where 'Ø' is the symbol produced when no signal is detected. Sifting: Alice and Bob broadcast their basis choices over the classical channel. We define the sets :={ i : a i = b i = ∧ y ′ i ≠Ø} and : { i : a i = b i = ∧ y ′ i ≠Ø}. The protocol repeats the first steps as long as either | |< n or | |< k . Parameter estimation : Alice and Bob choose a random subset of size n of and store the respective bits, y i and y ′ i , into raw key strings X and X ′, respectively. Next, they compute the average error where the sum is over all i ∈ . The protocol aborts if λ> Q tol . Error correction: An information reconciliation scheme that broadcasts at most leak EC bits of classical error correction data is applied. This allows Bob to compute an estimate, X̂ , of X . Then, Alice computes a bit string (a hash) of length by applying a random universal 2 hash function [46] to X . She sends the choice of function and the hash to Bob. If the hash of X̂ disagrees with the hash of X , the protocol aborts. Privacy amplification: Alice extracts ℓ bits of secret key S from X using a random universal 2 hash function [53] , [54] . (Instead of choosing a universal 2 hash function, which requires at least n bits of random seed, one could instead employ almost two-universal 2 hash functions [52] or constructions based on Trevisan's extractor [55] . These techniques allow for a reduction in the random seed length whereas the security claims remain almost unchanged.) The choice of function is communicated to Bob, who uses it to calculate Ŝ Security analysis The following two statements constitute the main technical result of our paper, stating that the protocols described above are both ɛ cor -correct and ɛ sec -secure, if the secret key length is chosen appropriately. Correctness is guaranteed by the error-correction step of the protocol, where a hash of Alice's raw key is compared with the hash of its estimate on Bob's side. The following holds: The protocols are ɛ sec -secure if the length of the extracted secret key does not exceed a certain length. Asymptotically for large block sizes n , the reductions of the key length due to finite statistics and security parameters can be neglected, and a secret key of length max = n ( q − h ( Q tol ))−leak EC can be extracted securely. Here h denotes the binary entropy function. Because our statistical sample is finite, we have to add to the tolerated channel noise a term that accounts for statistical fluctuations. Furthermore, the security parameters lead to a small reduction of the key rate logarithmic in ɛ cor and ɛ sec . The following holds: The protocol Φ [ n , k , , Q tol , ɛ cor , leak EC ] using a source with preparation quality q is ɛ sec -secret if the secret key length satisfies A sketch of the proof of these two statements follows in the methods section and a rigorous proof of slightly more general versions of the theorems presented above can be found in Supplementary Material 1 . In this section, we discuss the asymptotic behaviour of our security bounds and compare numerical bounds on the key rate for a finite number of exchanged signals with previous results. For this purpose, we assume that the quantum channel, in the absence of an eavesdropper, can be described as a depolarizing channel with quantum bit error rate Q . (This assumption is not needed for the security analysis of the previous section.) The numerical results are computed for a perfect single-photon source, that is, q =1. Furthermore, finite detection efficiencies and channel losses are not factored into the key rates, that is, the expected secret key rate calculated here can be understood as the expected key length per detected signal. The efficiency of a protocol Φ is characterized in terms of its expected secret key rate, where M ( n , k ) is the expected number of qubits that need to be exchanged until n raw key bits and k bits for parameter estimation are gathered (see protocol description). Before presenting numerical results for the optimal expected key rates for finite n , let us quickly discuss its asymptotic behaviour for arbitrarily large n . It is easy to verify that the key rate asymptotically reaches r max ( Q )=1−2 h ( Q ) for arbitrary security bounds ɛ >0. To see this, error correction can be achieved with a leakage rate of h ( Q ) (for example, see ref. 42 ). Furthermore, if we choose, for instance, k proportional to the statistical deviation in equation (2), μ , vanishes and the ratio between the raw key length, n , and the expected number of exchanged qubits, M ( n , k ), approaches one as n tends to infinity, that is, n / M ( n , k )→1. This asymptotic rate is optimal [43] . Finally, the deviations of the key length in equation (2) from its asymptotic limit can be explained as fluctuations that are due to the finiteness of the statistical samples we consider and the error bounds we chose. These terms are necessary for any finite-key analysis. In particular, one expects a statistical deviation μ that scales with the inverse of the square root of the sample size k as in equation (2) from any statistical estimation of the error rate. In this sense, our result is tight. To obtain our results for finite block sizes n , we fix a security bound ɛ and define an optimized ɛ -secure protocol, Φ * [ n , ɛ ], that results from a maximization of the expected secret key rate over all ɛ -secure protocols with block size n . For the purpose of this optimization, we assume an error correction leakage of leak EC = ξnh ( Q tol ) with ξ =1.1. Moreover, we bound the robustness ɛ rob by the probability that the measured security parameter exceeds Q tol , which (for depolarizing channels) decays exponentially in Q tol − Q . (For general quantum channels, the error rate in the and bases may be different. Hence, the error correction leakage is, in general, not a function of Q tol but of the expected error rate in the basis. Similarly, ɛ rob generally is the sum of the robustness of parameter estimation as above and the robustness of the error correction scheme. In this discussion, the analysis is simplified as we consider a depolarizing channel, and, thus, the expected error rate is the same in both bases.) In Fig. 1 , we present the expected key rates r = r ( Φ , Q ) of the optimal protocols Φ *[ n , ɛ ] as a function of the block size n . These rates are given for a fixed value of the security rate , that is, the amount by which the security bound ɛ increases per generated key bit. (In other words, can be seen as the probability of key leakage per key bit.) The plot shows that significant key rates can be obtained already for n =10 4 . 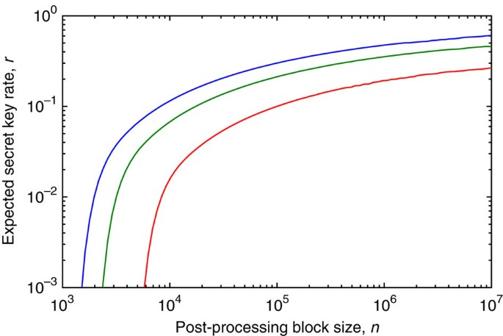Figure 1: Expected key rate as function of the block size. Plot of expected key rateras a function of the block sizenfor channel bit error ratesQ∈{1%, 2.5%, 5%} (from left to right). The security rate is fixed to=10−14. Figure 1: Expected key rate as function of the block size. Plot of expected key rate r as a function of the block size n for channel bit error rates Q ∈ {1%, 2.5%, 5%} (from left to right). The security rate is fixed to =10 −14 . Full size image In Table 1 , we provide selected numerical results for the optimal protocol parameters that correspond to block sizes n ={10 4 , 10 5 , 10 6 } and quantum bit error rates Q ∈ {1%, 2.5%}. These block sizes exemplify current hardware limitations in practical QKD systems. Table 1 Optimized parameters for security rate ɛ / ℓ =10 −14 . Full size table In Fig. 2 , we compare our optimal key rates with the maximal key rates that can be shown secure, using the finite key analysis of Scarani and Renner [18] . For comparison with previous work, we plot the rate ℓ / n , that is, the ratio between key length and block size, instead of the expected secret key rate as defined by equation (3). We show a major improvement in the minimum block size required to produce a provably secret key. The improvements are mainly due to a more direct evaluation of the smooth min-entropy via the entropic uncertainty relation and the use of statistics optimized specifically to the problem at hand ( Supplementary Note 2 ). 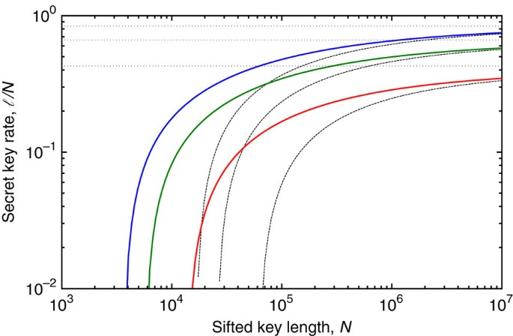Figure 2: Comparison of key rate with earlier results. The plots show the rateℓ/Nas a function of the sifted key lengthN=n+kfor various channel bit error ratesQ(as inFig. 1) and a security bound ofɛ=10−10. The (curved) dashed lines show the rates that can be proven secure using ref.18. The horizontal dashed lines indicate the asymptotic rates forQ∈{1%, 2.5%, 5%} (from top to bottom). Figure 2: Comparison of key rate with earlier results. The plots show the rate ℓ / N as a function of the sifted key length N = n + k for various channel bit error rates Q (as in Fig. 1 ) and a security bound of ɛ =10 −10 . The (curved) dashed lines show the rates that can be proven secure using ref. 18 . The horizontal dashed lines indicate the asymptotic rates for Q ∈ {1%, 2.5%, 5%} (from top to bottom). Full size image In conclusion, this article gives tight finite-key bounds for secure quantum key distribution with an asymmetric BB84 protocol. Our novel proof technique, based on the uncertainty principle, offers a conceptual improvement over earlier proofs that relied on a tomography of the state shared between Alice and Bob. Most previous security proofs against general adversaries [7] , [18] , [21] , [20] , are arranged in two steps: An analysis of the security against adversaries restricted to collective attacks and a lifting of this argument to general attacks. The lifting is often possible without a significant loss in key rate using modern techniques [24] , [25] ; hence, the main difference lies in the first part. In security proofs against collective attacks, Alice and Bob usually do tomography on their shared state, that is, they characterize the density matrix of their shared state. As the eavesdropper can be assumed to hold a purification of this state, it is then possible to bound the von Neumann entropy of the eavesdropper on Alice's measurement result. The min-entropy of the eavesdropper (which characterizes the probability of the eavesdropper guessing the secret key) is, in turn, bounded using the quantum asymptotic equipartition property [7] , [44] , introducing a penalty scaling with on the key rate. (A notable exception is [20] where the min-entropy is bounded directly from the results of tomography.) In contrast, our approach bounds the min-entropy directly and does not require us to do tomography on the state shared between Alice and Bob. In fact, we are only interested in one correlation (between Z and Z ′) and, thus, our statistics can be produced more efficiently. (However, that this is also the reason why our approach does not reach the asymptotic key rate for the six-state protocol [45] . There, full tomography puts limits on Eve's information that go beyond the uncertainty relation in ref. 22 .) Finally, as our considerations are rather general, we believe that they can be extended to other QKD protocols. Correctness The required correctness is ensured in the error-correction step of the protocol, when Alice and Bob compute a random hash function of their keys. If these hash values disagree, the protocol aborts and both players output empty keys (These keys are trivially correct.). Because arbitrary errors in the key will be detected with high probability when the hash values are compared [46] , we can guarantee that Alice's and Bob's secret keys are also the same with high probability. Secrecy To establish the secrecy of the protocols, we consider a gedankenexperiment in which Alice and Bob, after choosing a basis according to probabilities p x and p z as usual, prepare and measure everything in the basis. We denote the bit strings of length n that replace the raw keys X and X ′ in this hypothetical protocol as Z and Z ′, respectively. The secrecy then follows from the fact that, if Alice has a choice of encoding a string of n uniform bits in either the or basis, the following holds: the better Bob is able to estimate Alice's string if she prepared in the Z basis, the worse Eve is able to guess Alice's string, if she prepared in the basis. This can be formally expressed in terms of an uncertainty relation for smooth entropies [22] , where ɛ ≥0 is called a smoothing parameter and q , as seen below, is the preparation quality defined previously. The smooth min-entropy, ( X | E ), introduced in ref. 7 , characterizes the average probability that Eve guesses X correctly using her optimal strategy with access to the correlations stored in her quantum memory [47] . The smooth max-entropy, ( Z | Z ′), corresponds to the number of extra bits that are needed to reconstruct the value of Z using Z ′ up to a failure probability [48] . For precise mathematical definitions of the smooth min- and max-entropy, we refer to ref. 49 . The sources we consider in this article are either (a) qubit sources or (b) sources that create BB84 states by measuring part of an entangled state. In case b), a comparison with ref. 22 reveals that the bound on the uncertainty is given by −log c , where c is the overlap of the two measurement employed in the source. For general positive operator-valued measurements, { M x } for preparing in the basis and { N z } for preparing in the basis, this overlap is given by . This justifies the definition of the preparation quality q =−log c for such sources. In case a), the preparation process can be purified into an entanglement-based one of the type above. To see this, simply consider a singlet state between two qubits and projective measurements on the first qubit. It is easy to verify that the overlap of the prepared states in the two bases is equal to the overlap of the two projective measurements used to prepare them. Hence, the preparation quality of this source is given by q =−log c , where c is the maximum overlap of the prepared states. In the gedankenexperiment picture, the observed average error, λ , is calculated from k measurements sampled at random from n + k measurements in the basis. Hence, if λ is small, we deduce that, with high probability, Z and Z ′ are highly correlated and, thus, ( Z | Z ′) is small. In fact, as the protocol aborts if λ exceeds Q tol , the following bound on the smooth max-entropy (conditioned on the correlation test passing) holds: where μ takes into account statistical fluctuations and depends on the security parameter via Equation (5) is shown in Supplementary Note 2 , using an upper bound by Serfling [50] on the probability that the average error on the sample, λ , deviates by more than μ from the average error on the total string [51] . In addition to the uncertainty relation, our analysis employs the Quantum Leftover Hash Lemma [7] , [52] , which gives a direct operational meaning to the smooth min-entropy. It asserts that, using a random universal 2 hash function, it is possible to extract a Δ-secret key of length from X , where Here E′ summarizes all information Eve learned about X during the protocol, including the classical communication sent by Alice and Bob over the authenticated channel. For the protocol discussed here, a maximum of leak EC + ⌈ log(1/ ɛ cor ) ⌉ bits of information about X are revealed to the eavesdropper during the protocol. Hence, using a chain rule for smooth min-entropies, we can relate the smooth min-entropy before the classical post-processing, ( X | E ), with the min-entropy before privacy amplification, ( X | E ′) as follows. Collecting the bounds on the smooth entropies we got from the uncertainty relation, (4), and the parameter estimation, (5), we further find that Combining this with the Quantum Leftover Hashing Lemma (6) and using the bound on the key length given in equation (2), we get Finally, the protocol is ɛ sec -secret, if we choose ɛ proportional to ɛ sec and sufficiently small. How to cite this article: Tomamichel, M. et al . Tight finite-key analysis for quantum cryptography. Nat. Commun. 3:634 doi: 10.1038/ncomms1631 (2012).